Versatile control ofPlasmodium falciparumgene expression with an inducible protein–RNA interaction The available tools for conditional gene expression in Plasmodium falciparum are limited. Here, to enable reliable control of target gene expression, we build a system to efficiently modulate translation. We overcame several problems associated with other approaches for regulating gene expression in P. falciparum . Specifically, our system functions predictably across several native and engineered promoter contexts, and affords control over reporter and native parasite proteins irrespective of their subcellular compartmentalization. Induction and repression of gene expression are rapid, homogeneous and stable over prolonged periods. To demonstrate practical application of our system, we used it to reveal direct links between antimalarial drugs and their native parasite molecular target. This is an important outcome given the rapid spread of resistance, and intensified efforts to efficiently discover and optimize new antimalarial drugs. Overall, the studies presented highlight the utility of our system for broadly controlling gene expression and performing functional genetics in P. falciparum . Malaria is a disease caused by several species of Plasmodium parasites, and continues to be an enormous burden on global human health. Few preventative and treatment options are available. A key barrier to defining parasite vulnerabilities that can be targeted for therapeutic purposes has been the lack of a more complete genetic toolkit. For P. falciparum , the parasite responsible for the majority of human malaria deaths, the RNA interference strategy that has proven invaluable in other organisms is unavailable [1] . Conditional recombination to delete genes has been recently demonstrated [2] , but a generally applicable system for reversible regulation of gene expression remains highly sought. Methods to achieve robust transcriptional regulation remain elusive, although some attempts have been described [3] , [4] . A high degree of expression heterogeneity, and the unpredictable and rapid loss of regulatory behaviour have significantly limited their use in functional studies [3] , [5] . For these reasons, efforts to functionally regulate parasite genes, such as the P. falciparum chloroquine resistance transporter (PfCRT), using this approach were unsuccessful [5] . Recently, a modified version of this inducible transcription system has been described, and functional control of gene expression was achieved in the genetically tractable rodent model parasite, P. berghei [4] . However, functional regulation of gene expression in the more recalcitrant P. falciparum was not reported. In addition, although control of green fluorescent protein (GFP) reporter expression was assessed in P. falciparum , flow cytometry data on the cell-to-cell variability of this regulation is unavailable. Thus, it is unclear whether the key issues of heterogeneous expression and spontaneous loss of regulation observed specifically in P. falciparum have been resolved. From this perspective, the long-term reliability of existing inducible transcription systems in P. falciparum is unknown. An alternative system based on the inducible degradation of targeted proteins has been used effectively in some instances [6] , [7] . However, it is not generalizable to many genes, as the target protein must: (i) tolerate fusion to a ligand-sensitive degradation domain and (ii) be accessible to the parasite’s proteasome. This limits reliably performing functional studies on a substantial number of proteins that are trafficked to various subcellular compartments [8] , [9] , [10] and the host red blood cell (RBC) [11] . Recently, the glmS ribozyme has been used to post-transcriptionally control gene expression in P. falciparum [12] . However, together with the degradation domain system and its limitations described above, these comprise an extremely limited toolkit for achieving reversible control of gene expression in P. falciparum when compared with the many robust and orthogonal options available for regulating gene expression in other organisms. We previously engineered a system for inducible control of eukaryotic translation that uses a protein–RNA interaction controlled by a tetracycline analogue [13] ( Fig. 1a ). As the cytosolic translation machinery in P. falciparum is highly conserved with other eukaryotes [14] , we reasoned that we should be able to implement our system to control translation in the parasite. Three key attributes of this system are that it enables experimental control of gene expression independently of: (i) transcriptional control; (ii) modification of the target protein in a manner that potentially compromises its function and (iii) the specific compartment to which target proteins are trafficked. These satisfy important criteria for defining a broadly applicable gene regulatory system. Here we demonstrate implementation of our TetR-aptamer system to control both reporter and native gene expression in P. falciparum in a manner that meets the criteria outlined above. We also show that this system is useful for studying the function of native parasite genes. 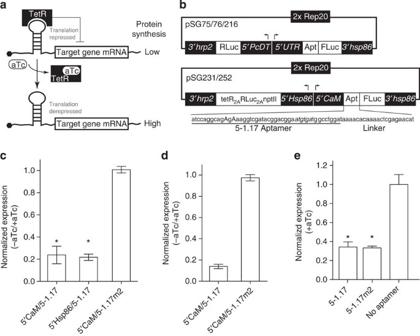Figure 1: Aptamer 5-1.17 enables aTc-dependent control of reporter gene expression. (a) A schematic of aTc- and TetR-dependent regulation of translation is shown. (b) Plasmid vectors pSG75 (CaM5′UTR with 5-1.17), pSG76 (CaM5′UTR with 5-1.17m2) and pSG216 (hsp865′UTR with 5-1.17) were used to screen for aTc-dependent regulation in transient transfections. Vectors pSG231 (5-1.17) and pSG252 (5-1.17m2) were used for the same purposes in stable episomal parasite lines. Either a functional (5-1.17) or mutated (5-1.17m2) aptamer was placed upstream of the FLuc reporter gene to regulate its expression. The sequence and placement context for the 5-1.17 aptamer is shown as an inset. The capitalized ‘A’s are mutated to ‘T’s to produce the non-functional 5-1.17m2. Bases initalicsindicate a short upstream start/stop, and those in bold indicate a productive start codon that is kept in frame with the downstream coding sequence (CDS) of interest. A CDS may carry its own initiation codon, or not, with no effect on expression or regulation by aTc.Renillaluciferase (RLuc) is expressed constitutively, and serves as a reference during quantification. (c) During transient screening in the TetR-expressing parasite clone B10, 5-1.17, but not 5-1.17m2, results in aTc-inducible FLuc expression. Values are expressed as FLuc/RLuc (–aTc) normalized to FLuc/RLuc (+aTc). (d) Similarly, in stable episomal lines, 5-1.17 but not 5-1.17m2, resulted in aTc-inducible FLuc expression. (e) Insertion of aptamer 5-1.17 downstream of theCaM5′UTR reduces its maximal FLuc expression about twofold. All data are expressed as the mean±s.d. of two to four independent experiments. An asterisk (*) denotes aP-value ≤0.002 determined by two-tailed unpairedt-test. Figure 1: Aptamer 5-1.17 enables aTc-dependent control of reporter gene expression. ( a ) A schematic of aTc- and TetR-dependent regulation of translation is shown. ( b ) Plasmid vectors pSG75 ( CaM 5′UTR with 5-1.17), pSG76 ( CaM 5′UTR with 5-1.17m2) and pSG216 ( hsp86 5′UTR with 5-1.17) were used to screen for aTc-dependent regulation in transient transfections. Vectors pSG231 (5-1.17) and pSG252 (5-1.17m2) were used for the same purposes in stable episomal parasite lines. Either a functional (5-1.17) or mutated (5-1.17m2) aptamer was placed upstream of the FLuc reporter gene to regulate its expression. The sequence and placement context for the 5-1.17 aptamer is shown as an inset. The capitalized ‘A’s are mutated to ‘T’s to produce the non-functional 5-1.17m2. Bases in italics indicate a short upstream start/stop, and those in bold indicate a productive start codon that is kept in frame with the downstream coding sequence (CDS) of interest. A CDS may carry its own initiation codon, or not, with no effect on expression or regulation by aTc. Renilla luciferase (RLuc) is expressed constitutively, and serves as a reference during quantification. ( c ) During transient screening in the TetR-expressing parasite clone B10, 5-1.17, but not 5-1.17m2, results in aTc-inducible FLuc expression. Values are expressed as FLuc/RLuc (–aTc) normalized to FLuc/RLuc (+aTc). ( d ) Similarly, in stable episomal lines, 5-1.17 but not 5-1.17m2, resulted in aTc-inducible FLuc expression. ( e ) Insertion of aptamer 5-1.17 downstream of the CaM 5′UTR reduces its maximal FLuc expression about twofold. All data are expressed as the mean±s.d. of two to four independent experiments. An asterisk (*) denotes a P -value ≤0.002 determined by two-tailed unpaired t -test. Full size image Regulatory system design and functional validation We used a plasmid-based transient screening approach to establish the basic functionality of our system in P. falciparum. We constructed a 3D7 parasite strain stably expressing TetR from a single-copy chromosomal locus ( Supplementary Fig. 1a,b and Supplementary Table 1 ), and transfected it with dual-luciferase reporter plasmids expressing firefly luciferase (FLuc) under the control of the TetR-binding aptamer 5-1.17, and a reference Renilla luciferase (RLuc; Fig. 1b ). Addition of anhydrotetracycline (aTc) to transiently transfected parasites yielded an ~80% change in FLuc expression ( Fig. 1c ), similar to what we observed in yeast [13] . This regulatory behaviour was consistent across different promoter/5′-untranslated region (5′UTR) contexts, with a similar dynamic range observed when regulating the hsp86 and calmodulin 5′UTRs. The mutant sequence 5-1.17m2, which does not interact with TetR [13] , yielded no aTc-dependent regulation, as expected. To further characterize this system, we built single plasmids expressing aptamer-regulated FLuc, a constitutive reference RLuc, TetR and a G418-selectable marker ( Fig. 1b ). These constructs express polycistronic messages that use 2A-like peptides to yield multiple distinct proteins [15] . A key benefit of this ‘all-in-one’ design is that it obviates the need for a dedicated TetR-expressing background line, and makes this system broadly useful in any P. falciparum strain of interest. We transfected single-plasmid constructs into parasite strain Dd2 and measured aTc-dependent luciferase expression after G418 selection. In this context, the system produced a similar ~80% regulation upon aTc addition ( Fig. 1d ). FLuc expression increased in a sigmoidal manner with aTc, reaching a maximum at an aTc concentration well below the minimum that inhibits parasite growth ( Supplementary Fig. 2a,b ). To establish that regulation occurs at the translational level, and not via a change in steady-state mRNA concentration, we measured FLuc mRNA by quantitative PCR ( Supplementary Fig. 3a ). We also verified by western blot analysis that aTc has no impact on TetR expression ( Supplementary Fig. 3b ). We observed that inclusion of the aptamer sequence (in the absence of TetR binding) decreased maximal FLuc expression possible from a given 5′UTR by about twofold compared to when no aptamer is present ( Fig. 1e ). Regulation dynamics during blood stage parasite development P. falciparum develops over a 48-h intraerythrocytic developmental cycle (IDC), during which individual genes are expressed in a temporally variable manner [16] , [17] . To best study the IDC, the TetR-aptamer system should allow rapid changes in target gene expression, with induction and washout times that are significantly less than a single IDC. We characterized aTc-dependent response kinetics in synchronized parasites expressing a stable 5-1.17–FLuc or 5-1.17m2–FLuc reporter ( Fig. 2 ). In one scenario, initially induced or repressed late schizont stage cultures (40 h post invasion) were washed, and each maintained thereafter in either the presence or absence of aTc over the next IDC ( Fig. 2a ). At 12 h post aTc addition, FLuc expression was indistinguishable from a culture continuously exposed to aTc. Repression after aTc washout was similarly rapid, and FLuc levels returned to basal repressed levels early into the IDC. In a second scenario, induction or washout was performed soon after invasion (early ring stage) and FLuc expression was monitored within the same IDC ( Fig. 2b ). The changes in expression were nearly complete at the first time point (5 h), although the apparent magnitude of FLuc repression after aTc washout was not as complete under these conditions. The inherent turnover rate of pre-synthesized FLuc protein, rather than TetR–aptamer interaction dynamics, is likely rate limiting and gives rise to the residual FLuc activity detected in the aTc washout phase of these experiments. Consistent with this interpretation, engineered mRNA and protein destabilizing signals are needed to improve the reliability of FLuc as a reporter of decreased protein synthesis in rapid kinetics studies [18] . 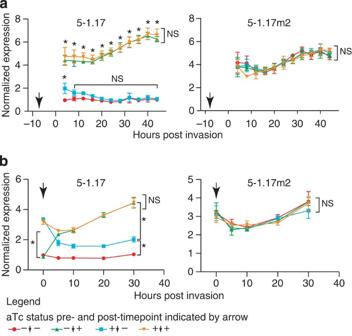Figure 2: Rapid induction and washout kinetics are achieved using the TetR-aptamer system inP. falciparum. Dd2 strain parasites harbouring pSG231 (5-1.17/FLuc) or pSG252 (5-1.17m2/FLuc) were tightly synchronized. aTc (1 μM) was added, removed or maintained at the time indicated by the arrowhead. Dual luciferase measurements were made at various time points, and relative FLuc/RLuc ratios were determined. (a) aTc status was adjusted in late-stage parasites just before reinvasion, and FLuc/RLuc monitored over the next IDC; (b) aTc status was adjusted at early ring stage, and FLuc/RLuc monitored within that IDC. Values represent the mean±s.d. of three biological replicates. An asterisk (*) denotes aP-value≤0.001 as determined by two-way analysis of variance. NS=not significant. Figure 2: Rapid induction and washout kinetics are achieved using the TetR-aptamer system in P. falciparum . Dd2 strain parasites harbouring pSG231 (5-1.17/FLuc) or pSG252 (5-1.17m2/FLuc) were tightly synchronized. aTc (1 μM) was added, removed or maintained at the time indicated by the arrowhead. Dual luciferase measurements were made at various time points, and relative FLuc/RLuc ratios were determined. ( a ) aTc status was adjusted in late-stage parasites just before reinvasion, and FLuc/RLuc monitored over the next IDC; ( b ) aTc status was adjusted at early ring stage, and FLuc/RLuc monitored within that IDC. Values represent the mean±s.d. of three biological replicates. An asterisk (*) denotes a P -value≤0.001 as determined by two-way analysis of variance. NS=not significant. Full size image Regulation in chromosomal context and of subcellular targets Towards adapting the TetR-aptamer system to regulate endogenous gene expression, we tested its regulatory performance using integrated reporter genes. We first integrated our single-plasmid attP + constructs ( Supplementary Fig. 4a,b ) at single copy into the chromosome at the cg6 locus of NF54-attB parasites [19] using the Bxb1 site-specific recombinase [20] . The expression of both luciferase and GFP reporters were regulated similarly (~80%) in this context ( Supplementary Fig. 5a ). In addition, the GFP reporter illustrated that both the repressed and induced parasite populations were homogeneously regulated ( Supplementary Fig. 5b ). Furthermore, aTc-dependent regulation is fully preserved with our system even after prolonged continuous culture (>8 months) in both episomal and integrated contexts. Significantly, this contrasts with a previously reported TetR-based transcriptional system where regulation was very heterogeneous and unpredictably short-lived [3] , [5] . We then examined the utility of our system to regulate the expression of genes targeted to various parasite subcellular organelles and the host RBC while preserving proper trafficking. To our GFP construct, we added N-terminal targeting peptides that mediate trafficking to the apicoplast [21] , mitochondrion [22] or host erythrocyte cytoplasm [23] , [24] downstream of the regulatory aptamer. As translation likely initiates within the aptamer [13] , it is important to establish that the aptamer-encoded short leader peptide does not interfere with target protein trafficking. Direct or indirect fluorescence microscopy of live or antibody-probed fixed cells, respectively, revealed that including the aptamer upstream of the subcellular targeting sequence did not interfere with proper protein trafficking ( Fig. 3a ). Flow cytometry analysis again confirmed that aTc-dependent induction of GFP expression is homogeneous in these strains ( Supplementary Fig. 5c ). The organelle-targeted GFP constructs yielded lower fluorescence signal. As the signal-to-noise ratio was too low to accurately quantify aTc-dependent changes in GFP expression by flow cytometry, we quantified GFP expression by ELISA ( Supplementary Fig. 5d ). This analysis revealed aTc-dependent regulation of GFP targeted to the apicoplast and mitochondrion is similar to that achieved during cytosolic expression. We further confirmed these findings using the native parasite exported protein knob-associated histidine-rich protein (KAHRP; PF3D7_0202000). This protein is exported to the host RBC and associates with the cytoskeletal network just beneath the RBC membrane, which results in a rim fluorescence pattern upon microscopy [25] , [26] . We constructed a P. falciparum centromere plasmid [27] from which GFP fused to KAHRP (KAHRP-GFP) [25] is expressed under the control of the native KAHRP upstream region (~2 kb) and regulated by aptamer 5-1.17. This plasmid uses the versatile ‘all-in-one’ design introduced earlier and also encodes the regulatory TetR, a constitutive luciferase and a selectable marker ( Supplementary Fig. 6a ). Parasites transfected with this KAHRP-GFP construct and induced with aTc displayed prominent GFP signal closely associated with the RBC plasma membrane, indicating the expected export and localization of this protein ( Fig. 3b ). Flow cytometric analysis comparing uninduced and aTc-induced parasites revealed an ~80% regulation in KAHRP-GFP expression level ( Supplementary Fig. 6b ). A low GFP expressing but aTc non-responsive sub-population observed during flow cytometry likely reflects heterogeneity arising from episomal expression [20] . Consistent with this interpretation, we always observe single peaks of GFP expression that shift homogenously in response to aTc when using strains in which the regulated reporter is chromosomally integrated ( Supplementary Fig. 5b,c ). 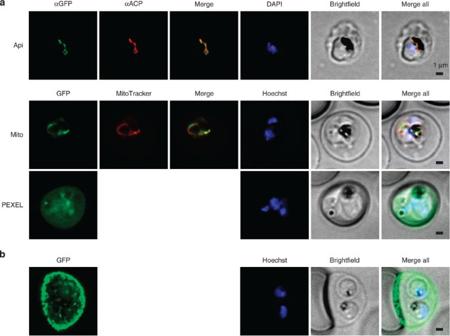Figure 3: Aptamer controlled target proteins are properly trafficked to various subcellular compartments. (a) Immunofluorescence and live fluorescence imaging of strains expressing chromosomally integrated GFP reporters bearing an N-terminal targeting peptide (Api=apicoplast-targeted; Mito=mitochondrion-targeted; PEXEL=protein export to erythrocyte cytoplasm). ACP=acyl carrier protein, used as an apicoplast marker. (b) Live fluorescence imaging of aptamer-regulated KAHRP-GFP fusion expressed from an episomal construct bearing theP. falciparumcentromere-derived elementpfCEN5–1.5. Figure 3: Aptamer controlled target proteins are properly trafficked to various subcellular compartments. ( a ) Immunofluorescence and live fluorescence imaging of strains expressing chromosomally integrated GFP reporters bearing an N-terminal targeting peptide (Api=apicoplast-targeted; Mito=mitochondrion-targeted; PEXEL=protein export to erythrocyte cytoplasm). ACP=acyl carrier protein, used as an apicoplast marker. ( b ) Live fluorescence imaging of aptamer-regulated KAHRP-GFP fusion expressed from an episomal construct bearing the P. falciparum centromere-derived element pfCEN5–1.5 . Full size image Regulating native gene expression to study function Next, we selected a second native parasite gene, the P. falciparum chloroquine (Cq) resistance transporter (PfCRT; PF3D7_0709000), to functionally regulate its expression and illustrate the utility of our system. The rationale for selecting this target was twofold in that PfCRT is: (i) trafficked to the parasite’s digestive vacuole and has been recalcitrant to functional regulation by existing methods [5] and (ii) an important antimalarial drug resistance determinant and target. We reasoned that establishing a validated line in which PfCRT expression is dynamically regulated would create an informative proof-of-concept model context, and serve as a useful reagent in future drug discovery efforts centred on interfering with PfCRT function. In this implementation, we also sought to demonstrate an efficient and generalizable strategy for installing regulatory TetR aptamers within a native chromosomal locus. This allows for dynamic control of target gene expression in isogenic parasite lines. We used a zinc finger nuclease (ZFN) targeting the PfCRT locus [28] to efficiently replace the Cq-sensitive allele (PfCRT 3D7 ) in 3D7 parasites with a resistant allele (PfCRT Dd2 ) regulated by the functional aptamer (5-1.17) or sham-regulated by the non-functional mutant (5-1.17m2; Fig. 4a ). The donor plasmids (pSG594/595) used to repair the ZFN-induced DNA double strand breaks were designed with a recoded PfCRT exon 1 to limit homology to the native locus. This ensures that repair initiated within the region homologous to the native 5′UTR is strongly favoured, and that the sequence encoding the aptamer is reliably introduced at the chromosomal locus. In addition, our donor plasmids are recoded at the ZFN cut site to ensure that chromosomal editing is irreversible. We co-transfected then co-selected for both ZFN and repair plasmids for 2 weeks, after which we selected only for the donor plasmid. Under these conditions, more than 50% of isolated clones were PCR positive for the desired integration outcome ( Supplementary Fig. 7 ), which is similar to the repair efficiency reported by Straimer et al . when using this ZFN pair to edit the PfCRT locus [28] . 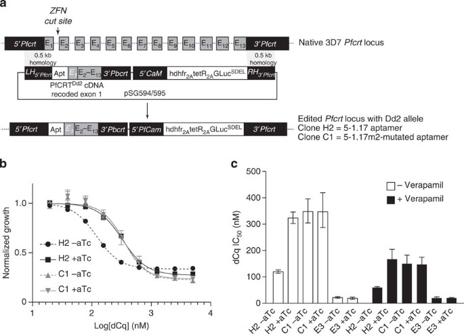Figure 4: Aptamer-mediated functional regulation of PfCRT expression from its native chromosomal context. (a) Schematic of modified PfCRT locus to simultaneously introduce the regulatory TetR protein, and either 5-1.17 (clone H2) or 5-1.17m2 (clone C1). (b) Aptamer 5-1.17 regulates the sensitivity of clone H2 to dCQ, whereas the non-functional 5-1.17m2 does not modulate the sensitivity of clone C1 to dCQ. (c) Verapamil (VP), which reverses resistance to dCQ through a direct interaction with PfCRT, is less effective when PfCRT expression is induced versus repressed. Clone E3 (control) has a wild-type PfCRT3D7locus and a constitutive GLucSDELreporter integrated at thecg6locus, and exhibits an aTc- and VP-independent IC50dCQ=20 nM (95% CI: 15–26 nM). Data were collected in biological triplicates. Mean values and error bars representing 95% confidence intervals are reported. Figure 4: Aptamer-mediated functional regulation of PfCRT expression from its native chromosomal context. ( a ) Schematic of modified PfCRT locus to simultaneously introduce the regulatory TetR protein, and either 5-1.17 (clone H2) or 5-1.17m2 (clone C1). ( b ) Aptamer 5-1.17 regulates the sensitivity of clone H2 to dCQ, whereas the non-functional 5-1.17m2 does not modulate the sensitivity of clone C1 to dCQ. ( c ) Verapamil (VP), which reverses resistance to dCQ through a direct interaction with PfCRT, is less effective when PfCRT expression is induced versus repressed. Clone E3 (control) has a wild-type PfCRT 3D7 locus and a constitutive GLuc SDEL reporter integrated at the cg6 locus, and exhibits an aTc- and VP-independent IC 50 dCQ =20 nM (95% CI: 15–26 nM). Data were collected in biological triplicates. Mean values and error bars representing 95% confidence intervals are reported. Full size image Both the aptamer and sham-regulated lines grew at approximately half the rate of the parental 3D7 strain. This could be due to a decrease in maximum PfCRT expression caused by the combined effect of aptamer insertion described earlier and replacement of the intron-containing allele with a cDNA-based one. Indeed, previous studies have shown that cDNA-based PfCRT Dd2 alleles are expressed at lower levels [29] and that decreased expression is associated with reduced growth relative to parental strains with intron-containing alleles [30] . Furthermore, although lines with a PfCRT Dd2 cDNA-based allele could readily be obtained in the GC03 genetic background that was derived in a cross between the CQ-sensitive HB3 and CQ-resistant Dd2 (ref. 31 ), attempts to generate this genotype in the CQ-sensitive 3D7 background by single crossover recombination were unsuccessful [32] . This suggests that a significant fitness cost is associated with expressing the PfCRT Dd2 cDNA allele in a 3D7 background, as used in our studies, and this likely also contributes to the growth defect in our derived lines. An extremely valuable step in drug target identification and validation is the ability to directly link the effect of a compound to its putative target. We examined the suitability of our system for this purpose by measuring parasite growth in the presence of desethylchloroquine (dCq), a potent Cq metabolite, when PfCRT expression is either repressed (−aTc) or induced (+aTc). We used dCq instead of Cq as mutant PfCRT alleles expressed on the Cq-sensitive 3D7 background become significantly resistant to dCq but not Cq, likely because additional genetic and/or epigenetic changes present in inherently resistant strains contribute to imparting high-level resistance to both Cq and dCq [32] . Consistent with this, we detected no increased resistance to Cq in any of our parasite lines expressing the PfCRT Dd2 allele. However, in experiments where dCq was used, and PfCRT Dd2 expression controlled by the active aptamer, aTc increased the IC 50 dCq from 120 nM (95% CI: 113–127 nM) to 324 nM (95% CI: 303–345 nM), as is expected when increasing the expression level of this drug resistance determinant ( Fig. 4b,c ). No aTc-dependent effect on dCq sensitivity was observed in the mutant aptamer line (IC 50 dCq =348 nM (−aTc); 95% CI: 305–396 nM and 347 nM (+aTc); 95% CI: 287–419 nM)). This rules out a direct interaction between dCq and aTc as the basis for the observations with the functional aptamer. Furthermore, as the functional aptamer and its non-functional control differ only in their non-coding region, the identical PfCRT protein component is made in both cases. Therefore, the observed phenotypes are not due to the production of functionally distinct PfCRT protein. We note here that some PfCRT Dd2 expression occurs in the repressed state, and this confers some basal resistance to dCq (IC 50 =120 nM) compared with the parental line (IC 50 =20 nM). This is consistent with our earlier data ( Fig. 1c,d ) showing that expression is substantially reduced but not completely abolished in the repressed state. We further illustrated the utility of the TetR-aptamer system in the drug target identification framework by determining the aTc-dependence of verapamil (VP)-mediated reversal of dCq resistance. VP directly interacts with PfCRT [33] to inhibit the efflux of toxic 4-aminoquinoline drugs, such as dCq, from the digestive vacuole. Thus, when PfCRT expression is reduced, a lower VP concentration should be required to re-sensitize parasites to dCq than when PfCRT expression is increased. Consistent with this model, VP almost completely reversed parasite resistance to dCq when PfCRT Dd2 expression in the aptamer-regulated line was repressed (IC 50 dCQ =60 nM (− aTc,+VP); 95% CI: 56–64 nM; Fig. 4c ). However, induction of PfCRT Dd2 expression significantly limited this reversal effect (IC 50 dCQ =167 nM (+aTc,+VP); 95% CI: 137–205 nM), and these parasites remained similarly resistant to dCq as uninduced parasites that were not VP treated ( Fig. 4c ). In mutant aptamer lines, VP increased dCQ sensitivity, but this was aTc-independent (IC 50 dCQ =150 nM (−aTc,+VP); 95% CI: 123–183 versus 167 nM (+aTc,+VP); 95% CI: 137–205 nM). Taken together, these data support a potentially generalizable strategy for using the TetR-aptamer system to modulate the expression level of pre-specified molecular determinants to probe their mechanistic role in parasite sensitivity/resistance to candidate or established antimalarial drugs. In summary, we have built and demonstrated a tool with broad utility for controlling gene expression in P. falciparum. Because this system functions reliably with no apparent dependence on parameters such as 5′UTR length or sequence, target gene sequence, or subcellular trafficking of the regulated protein, it represents a versatile addition to the malaria research toolset. In addition, unlike ribozyme-based systems where only the RNA component can be engineered to improve functionality, our system provides the opportunity to engineer both the RNA element and TetR protein component [34] to extend and improve regulatory behaviour. Last, given that our system is based on fundamental principles of eukaryotic translational regulation, we envision that it will be broadly applicable and easily adaptable to other pathogenic organisms for which robust tools for inducible gene expression are currently lacking. Molecular cloning Cloning was performed by standard restriction/ligation, yeast homologous recombination or Gibson assembly methods as described [15] . Unless otherwise noted, enzymes were from New England Biolabs and reagents were from Sigma-Aldrich, Research Products International, GoldBio Technology or Alfa Aesar. PCR amplification of parasite DNA was performed either directly on infected RBCs (diluted 1:50 into the reaction) or on purified DNA templates using Hemo KlenTaq mixed 15:1 (v:v) with PfuTurbo (Agilent). Plasmid DNA was prepared for transfection using Maxi Columns (Epoch Life Science) or the Xtra Midi Kit (Clontech). Plasmid DNA sequences and sources GenBank files for the constructs used in this study are provided as Supplementary Files . FLuc is wild-type firefly luciferase DNA carrying the K549E mutation for cytosolic targeting in yeast [35] . Green fluorescent protein is GFPmut2 (ref. 36 , cloned from pFGNr (Malaria Research and Reference Reagent Resource Center, MR4; http:// www.mr4.org ). P. falciparum culture and transfection Parasites were grown in human erythrocytes at 2% haematocrit under 5% O 2 and 5% CO 2 in RPMI 1640 media supplemented with 5 g l −1 of Albumax II (Life Technologies), 2 g l −1 of NaHCO 3 , 25 mM HEPES-K, pH 7.4, 1 mM hypoxanthine and 50 mg l −1 of gentamicin. Transfections used 25–75 μg of each plasmid per 200 μl packed RBC, adjusted to 50% haematocrit, and were performed by the spontaneous DNA uptake method [37] . Electroporation was performed on a Bio-Rad Gene Pulser II (Bio-Rad) with eight square-wave pulses of 365 V for 1 ms, separated by 100 ms. Transfected parasites were selected with 2.5 mg l −1 Blasticidin S, 5 nM WR9920 (Jacobus Pharmaceuticals) and/or 250 mg l −1 G418 beginning 4 days after transfection. In the case of Bxb1 -mediated integration, no selection was applied on the integrase-expressing plasmid. All chromosomally modified strains were confirmed by diagnostic PCR and sequencing of these products. Luciferase measurement Dual measurement of FLuc and coelenterazine-utilizing luciferases was performed either with the Dual Luciferase Assay (Promega) or with homemade reagents as described [13] . Single measurement of GLucSDEL was performed by adding one volume of sample to ten volumes of assay buffer (0.5 × PBS, 0.025% Nonidet P-40, 1 μg ml −1 coelenterazine). Luciferase intensity was measured on a GloMax 20/20 luminometer (Turner Biosystems) or a Spectramax L plate reader (Molecular Devices). Minimum signals obtained using transient and stably transfected lines were ≥5-fold and ≥10 3 -fold above background, respectively, and within instrumentation linear response ranges. Flow cytometry Late-stage infected RBCs were enriched with a MACS LD column (Miltenyi Biotec) and stained for nucleic acid content with 1 μM SYTO 61 (Life Technologies) before analysis on an Accuri C6 flow cytometer (BD Biosciences). GFP was analysed in FL1-H and SYTO 61 in FL4-H. Parasites were gated on high FL4 intensity to eliminate contaminating uninfected RBCs. Addition of aTc to either uninfected or non-fluorescent-infected RBCs had no effect on FL1-H intensity. GFP ELISA Late-stage infected RBCs were enriched with a MACS LD column (Miltenyi Biotec) and RBC membranes were lysed with 0.5 g l −1 saponin in PBS. Parasites were washed repeatedly with PBS to remove visibly detectable haemoglobin and stored at −80 °C. As haemoglobin-depleted parasite fractions were analysed, KAHRP-targeted GFP was not analysed by this method. Parasite lysates were prepared and GFP content was analysed with the GFP ELISA kit (Abcam, ab117992). Wells were loaded with equal amounts of total extracted protein as determined by BCA protein assay (Thermo Scientific). GFP − 3D7 parasites were used as a background control and to establish that the inclusion of aTc did not affect background signal intensity. Sample preparation for immunofluorescent microscopy Late-stage infected RBCs were prepared by a method modified from Gallagher et al . [38] Cells were pelleted and resuspended in fixation solution (PBS+4% formaldehyde+4% glutaraldehyde) at 0.2% haematocrit. Fixation solution was prepared fresh from reagents in methanol-free ampules. Cells were immediately spotted onto polyethyleneimine-coated glass slides and incubated at room temperature for 30 min. An Immunopen (EMD Biosciences) was used to contain the cell suspension in a small droplet. Attached cells were washed with PBS and permeablized by incubating in 1% Triton X-100 in PBS for 10 min. Cells were then washed with PBS and blocked/quenched with 3% bovine serum albumin and 150 mM glycine in PBS for 1 h. Cells were probed with mouse monoclonal anti-GFP (12A6, 1:25) and rabbit anti-ACP (1:500) in 3% BSA in PBS at 4 °C overnight, washed with PBS, and probed with CF488A-conjugated donkey anti-mouse (Biotium, 20014-1, 1:1,000) and CF647-conjugated goat anti-rabbit (Biotium, 20282-1, 1:1,000) for 1 h at room temperature in the dark. Slides were washed with PBS and a #1.5 coverslip was mounted with ProLong Gold and 4',6-diamidino-2-phenylindole (Life Technologies) followed by incubation in the dark for at least 12 h before sealing and imaging. The GFP monoclonal antibody 12A6, developed by P.J. Sanchez, K.J. Daniels and D.R. Soll, was obtained from the Developmental Studies Hybridoma Bank, under the auspices of the Eunice Kennedy Shriver National Institute of Child Health and Human Development and maintained by the University of Iowa, Department of Biology, Iowa, IA, USA. Sample preparation for live fluorescence microscopy Late-stage infected RBC cultures were resuspended in Albumax-free growth media and attached to polyethyleneimine-coated glass-bottom dishes (MatTek) before staining for 30 min with 2 μg ml −1 Hoechst 33342 (Life Technologies), washing and resuspension in Opti-Klear imaging buffer (Marker Gene Technologies). For mitochondrial staining, cultures were incubated at 37 °C for 15 min in growth media containing 25 nM MitoTracker Deep Red FM (Life Technologies) before attachment. Fluorescence microscopy Imaging was performed on a Zeiss Axio Observer microscope (Zeiss) with a × 100 objective. For each field, a 30-image Z-stack was deconvolved with Huygens Essential software (SVI). Maximum intensity Z-projections, false colouring and image merging were performed with ImageJ software [39] . Quantitative PCR Quantitative PCR was performed as described [13] with PrimeTime 5′ nuclease assays (Integrated DNA Technologies). P. falciparum RNA was extracted directly from late-stage infected RBCs with Trizol (Life Technologies) and purified with an RNeasy kit (Qiagen). cDNA was prepared with SuperScript III reverse transcriptase (Life Technologies). PF3D7_1331700 ( glutamine-tRNA ligase ) was used as a housekeeping reference gene. Primer and probe sequences are listed in Supplementary Table 2 . ZFN-mediated editing of the PfCRT locus Parasites were co-transfected with ZFN-expressing plasmid (expressing blasticidin resistance) and a donor vector (expressing WR99210 resistance). Four days after transfection, cultures were selected with 2.5 mg l −1 blasticidin and 2.5 nM WR99210 for 2 weeks, at which point blasticidin selection was removed. During transfection and routine culturing, parasites were always maintained in the presence of 0.4 μM aTc. ATc was only removed as needed for specific experiments. Proper repair of the PfCRT locus with aptamer integration was confirmed by PCR in bulk culture and after cloning by limiting dilution. Greater than 50% of the clones isolated were PCR positive for the integration event. Drug toxicity assays Parasite growth in the presence or absence of antimalarial drugs was monitored with the Gaussia luciferase reporter GLucSDEL. The full-length Gaussia luciferase (human codon-optimized, New England Biolabs) was fused at its C terminus to the endoplasmic retention signal peptide SDEL, yielding extremely high coelenterazine-dependent luciferase reporter activity in P. falciparum. The high activity and stability of GLucSDEL allow monitoring of luciferase activity in the culture supernatant. For drug toxicity assays, synchronous ring-stage cultures were seeded in 96-well plates at 0.5% haematocrit and ~0.5% parasitemia. Serial dilutions of dCq (Santa Cruz Biotech) were added to a final concentration of 0 or 19.5–5,000 nM and cultures were incubated for 96 h. When applicable, VP (Enzo Life Sciences) was used at 0.8 μM. Plates were briefly centrifuged and 20 μl of culture supernatant was assayed for Gaussia luciferase activity as described above. Each experiment was performed in triplicate, and the positions of each condition (different strains and aTc induction conditions) were systematically varied to eliminate position bias. Luciferase-null background signal (from strain 3D7) was subtracted and luciferase intensities were normalized to the no drug conditions. IC 50 values and 95% confidence intervals were determined by nonlinear regression with Prism software (GraphPad). How to cite this article: Goldfless, S. J. et al . Versatile control of Plasmodium falciparum gene expression with an inducible protein–RNA interaction. Nat. Commun. 5:5329 doi: 10.1038/ncomms6329 (2014). Accession codes . Annotated sequence files for the plasmids used in this study are deposited in NCBI GenBank under accession codes: KM288848 ;(pSG58) KM288849 ;(pSG75) KM288850 ;(pSG76) KM288851 ;(pSG217) KM288852 ;(pSG230) KM288853 ;(pSG231) KM288854 ;(pSG252) KM288855 ;(pSG460) KM288856 ;(pSG463) KM288857 ;(pSG584) KM288858 ;(pSG586) KM288859 ;(pSG590) KM288860 ;(pSG594) KM288861 ;(pSG595) KM288862 (pSG594 with modified PF3D7_0709000 locus); KM288863 ; (pSG599) KM288864 ;(pSG600) KM288865 ;(pSG601) KM288866 ;(NF54_pSG479::pSG593) and KM288867 (annotated PF3D7_0709000 locus).